Thymic stromal lymphopoietin induces corticosteroid resistance in natural helper cells during airway inflammation Type-2 innate immune responses that occur in airways and are accompanied by goblet-cell hyperplasia and mucus production are largely driven by interleukin-33 (IL-33) and natural helper (NH) cells, a member of group 2 innate lymphoid cells (ILC2s) and the major target of IL-33. Here we report that the corticosteroid resistance observed as a result of airway inflammation triggered by sensitization and exposure to allergen is induced via the IL-33/NH-cell axis. Thymic stromal lymphopoietin (TSLP) synthesized during airway inflammation plays a pivotal role in the induction of NH-cell corticosteroid resistance in vitro and in vivo , by controlling phosphorylation of STAT5 and expression of Bcl-xL in NH cells. Blockade of TSLP with a neutralizing antibody or blocking the TSLP/STAT5 signalling pathway with low molecular-weight STAT5 inhibitors such as pimozide restores corticosteroid sensitivity. Thus, the TSLP-STAT5 pathway could be a new therapeutic target in severe, corticosteroid-resistant asthma. Asthma is a chronic airway disease characterized by persistent eosinophilic inflammation in the airways that is dependent on type-2 cytokines such as interleukin (IL)-5 and IL-13. As corticosteroids suppress the recruitment and activation of inflammatory cells, inhibit the expression of cytokines and chemokines, and attenuate airway inflammation, these are the key drugs for the treatment of asthma regardless of the atopic status or the presence of specific IgE responses to allergens [1] , [2] , [3] . Most asthma patients can be well controlled with a low-to-moderate dose of inhaled corticosteroids. However, about 5–10% of asthmatic patients respond poorly to a maximal dose of inhaled corticosteroids exhibiting sustained inflammatory cell infiltration in the airways [4] . In such patients with so-called ‘severe asthma’ or ‘refractory asthma’, uncontrolled and frequently exacerbated asthmatic symptoms profoundly impair their quality of life and also have a strong impact on health-care costs. Therefore, elucidating the mechanism of corticosteroid resistance in these patients is critical in the development of a highly effective, novel pharmacotherapy. Recent studies have demonstrated that an IL-1 family cytokine, IL-33 (ref. 5 ), is relevant to the pathophysiology of severe asthma. Single-nucleotide polymorphisms in the genes of IL-33 and T1/ST2, a receptor for IL-33, are associated with severe asthma [6] , [7] . IL-33 immunoreactivity in the airway smooth muscles cells is enhanced in the patients with severe asthma [8] . IL-33 can induce robust type-2 immune responses, eosinophilic inflammation and hyperresponsiveness in the airways independently of acquired immune system components, mast cells and basophils [9] . We previously identified natural helper (NH) cells [10] , a member of group 2 innate lymphoid cells (ILC2s) [11] , [12] , [13] , [14] , in fat-associated lymphoid clusters (FALC) [10] of adipose tissue. NH cells can produce large amounts of type-2 cytokines such as IL-5 and IL-13 in response to IL-33. Several groups have characterized populations of type-2 cytokine-producing ILCs associated with IL-33 mediate diseases in the lung [15] , [16] , [17] , [18] , [19] , [20] , [21] . However, it is unknown whether NH cells are involved in the observed corticosteroid sensitivity. In the present study, we reveal that IL-33 in the allergen-exposed airways induces accumulation of corticosteroid-resistant NH cells, type-2 cytokine production, airway inflammation and mucus production. We identify thymic stromal lymphopoietin (TSLP), which is highly expressed in the bronchial epithelium of the patients with severe asthma [22] , as a key cytokine that induces corticosteroid resistance in NH cells in vitro and in vivo , and demonstrate that blockade of TSLP or its signalling through STAT5 can restore corticosteroid sensitivity. Corticosteroid suppresses IL-33-induced airway inflammation IL-33 is a potent activator of NH cells [10] . Intranasal administration of IL-33 (1 μg per animal) for 3 consecutive days in C57BL/6 mice ( Fig. 1a ) causes a significant increase in the number of eosinophils in bronchoalveolar lavage fluid (BALF) ( Fig. 1b ) and NH cells in the lungs ( Fig. 1c ). NH cells are identified as lineage (CD4, CD5, CD8, CD19, NK1.1, CD11b, CD11c, FcεRI, B220, Gr-1 and TER119)-negative, Thy1 + c-Kit + Sca-1 + CD25 + IL-7R + ST2 dim cells ( Fig. 1d , Supplementary Fig. S1 ). Lung NH cells are more potent in producing IL-5 and IL-13 compared with CD4 + T cells, which are also increased in the lung in this model ( Fig. 1e ). 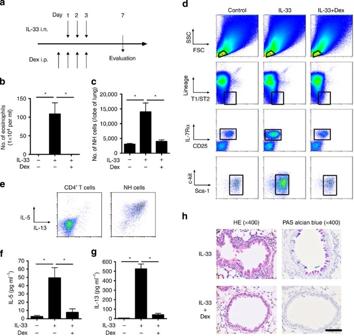Figure 1: Corticosteroids attenuate IL-33-induced airway inflammation and NH-cell accumulation. (a) Airway inflammation was induced with administration for 3 consecutive days of IL-33 (1 μg per animal, intranasal) in C57BL/6 mice. Dexamethasone (Dex, 5 mg kg−1) was injected intraperitoneally at 24 and 1 h before IL-33 administration for some mice. (b,c) Number of eosinophils in the BALF (b) and NH cells in the lungs (c) 4 days after the final administration of IL-33 or vehicle (PBS). Lung NH cells were counted as Lin−IL-7R+CD25+c-Kit+Sca-1+ST2dimcells. Mean±s.e.m.,n=3 for each group. *P<0.05 (Student’st-test) (d) Flow cytometric analysis of NH cells in the lung. (e) Intracellular staining of IL-5 and IL-13 in CD4+T cells and NH cells. (f,g) Amounts of IL-5 (f) and IL-13 (g) in the BALF were measured by ELISA. Mean±s.e.m.,n=3 for each group. *P<0.05 (Student’st-test). (h) Histology of airways from these mice stained with hematoxylin and eosin (left panels) or periodic acid–Schiff (PAS)-alcian blue (right panels). Scale bar, 100 μm. Data are representatives of three independent experiments. Figure 1: Corticosteroids attenuate IL-33-induced airway inflammation and NH-cell accumulation. ( a ) Airway inflammation was induced with administration for 3 consecutive days of IL-33 (1 μg per animal, intranasal) in C57BL/6 mice. Dexamethasone (Dex, 5 mg kg −1 ) was injected intraperitoneally at 24 and 1 h before IL-33 administration for some mice. ( b , c ) Number of eosinophils in the BALF ( b ) and NH cells in the lungs ( c ) 4 days after the final administration of IL-33 or vehicle (PBS). Lung NH cells were counted as Lin − IL-7R + CD25 + c-Kit + Sca-1 + ST2 dim cells. Mean±s.e.m., n =3 for each group. * P <0.05 (Student’s t -test) ( d ) Flow cytometric analysis of NH cells in the lung. ( e ) Intracellular staining of IL-5 and IL-13 in CD4 + T cells and NH cells. ( f , g ) Amounts of IL-5 ( f ) and IL-13 ( g ) in the BALF were measured by ELISA. Mean±s.e.m., n =3 for each group. * P <0.05 (Student’s t -test). ( h ) Histology of airways from these mice stained with hematoxylin and eosin (left panels) or periodic acid–Schiff (PAS)-alcian blue (right panels). Scale bar, 100 μm. Data are representatives of three independent experiments. Full size image Dexamethasone at a dose of 5 mg kg −1 body weight completely suppresses the IL-33-induced accumulation of eosinophils and lung NH cells ( Fig. 1b,c ), IL-5 and IL-13 production in the lungs ( Fig. 1f,g ), and peribronchial eosinophil accumulation and goblet-cell hyperplasia ( Fig. 1h ). It has been reported that IL-25 induces corticosteroid resistance through the induction of type-2 myeloid cells [23] , but IL-33 has only a marginal effect on type-2 myeloid cells compared with IL-25 ( Supplementary Fig. S2 ). As previously reported [24] , [25] , the same dose of dexamethasone suppresses eosinophil infiltration, synthesis of type-2 cytokines and mucous production in the airways of ovalbumin (OVA)-sensitized and challenged animals (OVA asthma model, Supplementary Fig. S3 ). These results suggest that both innate and acquired type-2 immune responses can be suppressed by corticosteroids. Corticosteroid resistance in an allergen+IL-33 inflammation We next examined the corticosteroid resistance when IL-33 was utilized in the OVA asthma model. To this end, we administered a low dose of IL-33 (0.1 μg per animal) to OVA asthma mice (OVA+IL-33, Fig. 2a ). At this dose, IL-33 causes little inflammation in the airways (5.7±1.3 versus 110±30 × 10 4 eosinophils per ml BALF in the animals administered with low (0.1 μg per animal) and high (1 μg per animal) dose of IL-33, respectively). In the OVA+IL-33 model, the increase in the number of lung NH cells ( Fig. 2c ) is equivalent to that induced by high-dose IL-33 (1 μg per animal, Fig. 1c ), whereas OVA exposure alone in sensitized animals does not increase the number of lung NH cells ( Supplementary Fig. S3c ). 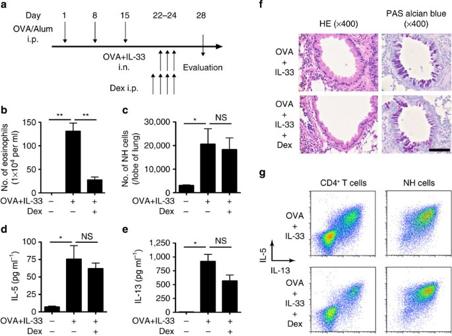Figure 2: Addition of IL-33 treatment to OVA asthma model mice. (a) OVA+IL-33-induced asthma model mice were treated by administration for 3 consecutive days of OVA (10 ng) and IL-33 (0.1 μg). The mice had been sensitized with OVA and alum. Dexamethasone (5 mg kg−1) was intraperitoneally injected at 24 and 1 h before OVA/IL-33 administration for some mice. (b,c) Number of eosinophils in the BALF (b) and NH cells in the lungs (c) 4 days after the final administration of OVA/IL-33 or vehicle (PBS). Mean±s.e.m.,n=3–4 for each group. NS, not significant. *P<0.05, **P<0.01 (Student’st-test). (d) Amounts of IL-5 (d) and IL-13 (e) in the BALF. Mean±s.e.m.,n=3–4 for each group. NS, not significant. *P<0.05 (Student’st-test). (f) Histology of the airways from these mice stained with hematoxylin and eosin (left panels) or periodic acid–Schiff (PAS)-alcian blue (right panels). Scale bar, 100 μm. (g) Intracellular staining of IL-5 and IL-13 in CD4+T cells and NH cells. Data are representatives of three independent experiments. Figure 2: Addition of IL-33 treatment to OVA asthma model mice. ( a ) OVA+IL-33-induced asthma model mice were treated by administration for 3 consecutive days of OVA (10 ng) and IL-33 (0.1 μg). The mice had been sensitized with OVA and alum. Dexamethasone (5 mg kg −1 ) was intraperitoneally injected at 24 and 1 h before OVA/IL-33 administration for some mice. ( b , c ) Number of eosinophils in the BALF ( b ) and NH cells in the lungs ( c ) 4 days after the final administration of OVA/IL-33 or vehicle (PBS). Mean±s.e.m., n =3–4 for each group. NS, not significant. * P <0.05, ** P <0.01 (Student’s t -test). ( d ) Amounts of IL-5 ( d ) and IL-13 ( e ) in the BALF. Mean±s.e.m., n =3–4 for each group. NS, not significant. * P <0.05 (Student’s t -test). ( f ) Histology of the airways from these mice stained with hematoxylin and eosin (left panels) or periodic acid–Schiff (PAS)-alcian blue (right panels). Scale bar, 100 μm. ( g ) Intracellular staining of IL-5 and IL-13 in CD4 + T cells and NH cells. Data are representatives of three independent experiments. Full size image In the OVA+IL-33 model, corticosteroid sensitivity is significantly reduced; dexamethasone treatment does not fully decrease the number of eosinophils ( Fig. 2b ), and fails to suppress the accumulation of lung NH cells ( Fig. 2c ), type-2 cytokine production ( Fig. 2d,e ) and mucus production in the bronchial epithelium ( Fig. 2f ). Importantly, IL-5/IL-13 production in NH cells is more resistant to the treatment with dexamethasone than in CD4 + T cells ( Fig. 2g , Supplementary Fig. S4 ). Collectively, the combination of innate and acquired type-2 immune responses induces corticosteroid resistance in airway inflammation along with lung NH cells. Corticosteroid sensitivity of NH cells The above results suggest that NH cells are resistant to corticosteroid. However, NH cells isolated from FALC are sensitive to corticosteroid: dexamethasone (10 −9 –10 −6 M) efficiently suppresses the proliferation of NH cells induced by IL-33 or a combination of IL-2 and IL-25 in a dose-dependent manner ( Fig. 3a ). A similar dose-dependency is observed in the ratio of dead cells/total cells; cell death is accelerated with corticosteroid regardless of the presence of IL-33 at a higher concentration (100 ng ml −1 ) ( Fig. 3b ). 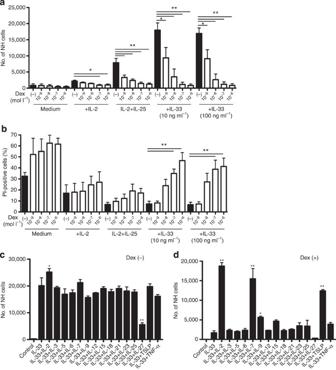Figure 3: Screening of cytokines that modify the corticosteroid sensitivity of NH cells. (a,b) NH cells (5,000 cells per well) derived from FALC were cultured with IL-2 (10 ng ml−1), IL-2+IL-25 (10 ng ml−1) or IL-33 (10 or 100 ng ml−1) in the presence or absence of dexamethasone (10−9–10−6M) for 4 days. Numbers of propidium iodide (PI)-negative cells (a) and the ratio of PI-positive cells among total cells (b) were determined using flow cytometry. Mean±s.e.m.,n=3 for each group. *P<0.05, **P<0.01 (ANOVA, Dunnet).P-values were presented as compared with no dexamethasone. (c,d) Number of PI-negative NH cells cultured with IL-33 (10 ng ml−1) and various cytokines (10 ng ml−1) for 4 days in the absence (c) or presence (d) of dexamethasone (10−8M). Mean±s.e.m.,n=3 for each group. *P<0.05, **P<0.01 (ANOVA, Dunnet).P-values were presented as compared with IL-33 alone. Data are representatives of three independent experiments. Figure 3: Screening of cytokines that modify the corticosteroid sensitivity of NH cells. ( a , b ) NH cells (5,000 cells per well) derived from FALC were cultured with IL-2 (10 ng ml −1 ), IL-2+IL-25 (10 ng ml −1 ) or IL-33 (10 or 100 ng ml −1 ) in the presence or absence of dexamethasone (10 −9 –10 −6 M) for 4 days. Numbers of propidium iodide (PI)-negative cells ( a ) and the ratio of PI-positive cells among total cells ( b ) were determined using flow cytometry. Mean±s.e.m., n =3 for each group. * P <0.05, ** P <0.01 (ANOVA, Dunnet). P -values were presented as compared with no dexamethasone. ( c , d ) Number of PI-negative NH cells cultured with IL-33 (10 ng ml −1 ) and various cytokines (10 ng ml −1 ) for 4 days in the absence ( c ) or presence ( d ) of dexamethasone (10 −8 M). Mean±s.e.m., n =3 for each group. * P <0.05, ** P <0.01 (ANOVA, Dunnet). P -values were presented as compared with IL-33 alone. Data are representatives of three independent experiments. Full size image Based on these findings, we hypothesized that some factors in the inflammatory milieu of the allergen-exposed airways induced the corticosteroid resistance in NH cells synergistically with IL-33. We therefore examined a panel of cytokines including IL-2, IL-3, IL-5, IL-6, IL-7, IL-9, IL-12, IL-15, IL-18, IL-21, IL-23, IL-25, IL-27, TSLP and TNF-α (tumour necrosis factor-α). In the absence of corticosteroids, IL-2 increases the IL-33-mediated NH-cell proliferation, whereas IL-27 suppresses it ( Fig. 3c ). In the presence of dexamethasone (10 −8 M), IL-2, IL-7, IL-9 or TSLP significantly increase the number of NH cells, or protect NH cells from corticosteroid effects ( Fig. 3d ), suggesting that these cytokines can induce corticosteroid resistance in NH cells. TSLP is associated with corticosteroid resistance in vivo Previous studies have revealed the involvement of TSLP in the patients with severe asthma as well as mouse asthma models [22] , [26] , [27] . Indeed, levels of Tslp mRNA and TSLP protein are elevated in the lungs of OVA alone or OVA+IL-33 model mice ( Supplementary Fig. S5 ). Furthermore, NH cells are more resistant to corticosteroid treatment than CD4 + T cells, which is possibly due to the higher expression of TSLPR in NH cells ( Supplementary Fig. S6 ). Administration of a neutralizing anti-TSLP antibody ( Fig. 4a ), which does not change the number of eosinophils or NH cells in OVA+IL-33 model without dexamethasone treatment ( Supplementary Fig. S7 ), significantly decreases the number of eosinophils in the BALF and the number of NH cells in the lung ( Fig. 4b,c ) as well as type-2 cytokine induction ( Fig. 4d,e ) synergistically with dexamethasone. Airway inflammation and goblet-cell hyperplasia are also significantly reduced by anti-TSLP antibody treatment ( Fig. 4f ), accompanied by a modest effect on the airway hyperresponsiveness ( Supplementary Fig. S8 ). In contrast, similar treatments with an anti-IL-2 or anti-IL-7 antibody, by itself or in combination with an anti-TSLP antibody, have little inhibitory effects on the number of eosinophils and lung NH cells in vivo ( Supplementary Fig. S9 ). 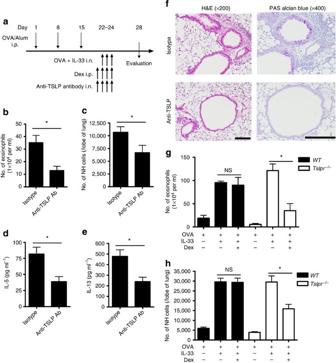Figure 4: An anti-TSLP antibody ameliorates corticosteroid resistance in an OVA plus IL-33-induced asthma model. (a) OVA, IL-33 and dexamethasone (5 mg kg−1) were administered to OVA-sensitized mice in combination with an anti-TSLP antibody (25 μg) or an isotype control antibody. (b,c) Number of eosinophils in the BALF (b) and NH cells in the lungs (c) 4 days after the final administration of OVA/IL-33/Dex/antibodies. Mean±s.e.m.,n=4 for each group. *P<0.05 (Student’st-test). (d,e) Concentrations of IL-5 (d) and IL-13 (e) in the BALF were measured by ELISA. Mean±s.e.m.,n=4 for each group. *P<0.05 (Student’st-test). (f) Representative histology of airways stained with hematoxylin and eosin (left panels) or periodic acid–Schiff (PAS)-alcian blue (right panels). Scale bar, 200 μm. (g,h) Number of eosinophils in the BALF (g) and NH cells in the lung (h) in wild-type (WT) andTslpr−/−mice sensitized with and exposed to OVA with or without IL-33 (0.1 μg) and/or dexamethasone (5 mg kg−1). Mean±s.e.m.,n=3–6 for each group. NS, not significant. *P<0.05 (Student’st-test). Data are representatives of three independent experiments. Figure 4: An anti-TSLP antibody ameliorates corticosteroid resistance in an OVA plus IL-33-induced asthma model. ( a ) OVA, IL-33 and dexamethasone (5 mg kg −1 ) were administered to OVA-sensitized mice in combination with an anti-TSLP antibody (25 μg) or an isotype control antibody. ( b , c ) Number of eosinophils in the BALF ( b ) and NH cells in the lungs ( c ) 4 days after the final administration of OVA/IL-33/Dex/antibodies. Mean±s.e.m., n =4 for each group. * P <0.05 (Student’s t -test). ( d , e ) Concentrations of IL-5 ( d ) and IL-13 ( e ) in the BALF were measured by ELISA. Mean±s.e.m., n =4 for each group. * P <0.05 (Student’s t -test). ( f ) Representative histology of airways stained with hematoxylin and eosin (left panels) or periodic acid–Schiff (PAS)-alcian blue (right panels). Scale bar, 200 μm. ( g , h ) Number of eosinophils in the BALF ( g ) and NH cells in the lung ( h ) in wild-type (WT) and Tslpr −/− mice sensitized with and exposed to OVA with or without IL-33 (0.1 μg) and/or dexamethasone (5 mg kg −1 ). Mean±s.e.m., n =3–6 for each group. NS, not significant. * P <0.05 (Student’s t -test). Data are representatives of three independent experiments. Full size image Although TSLP is a critical cytokine in the development of asthma in the OVA model [26] , the combination of OVA sensitization/exposure and IL-33 induces a robust eosinophilic inflammation in Tslpr −/− mice with a magnitude equivalent to that observed in wild-type mice ( Fig. 4g ). Interestingly, Tslpr −/− mice are more sensitive to dexamethasone than wild-type mice, and show a significant reduction in the number of BALF eosinophils and lung NH cells ( Fig. 4g,h ). In chimeric mice generated by transplantation of bone marrow cells from wild-type (CD45.2) and Tslpr −/− (CD45.1) congenic mice, Tslpr −/− NH cells tend to be more sensitive to dexamethasone treatment than wild-type cells during airway inflammation by OVA+IL-33 ( Supplementary Fig. S10 ). These results indicate that corticosteroid resistance is not induced efficiently in the absence of TSLP action. TSLP inhibits the corticosteroid-induced NH-cell apoptosis We next examined the role of TSLP in the corticosteroid resistance of NH cells derived from FALC and lung in vitro ( Fig. 5 ). Although dexamethasone strongly suppresses proliferation and type-2 cytokine production of NH cells in response to IL-33, TSLP mitigates the effects of corticosteroids on NH-cell proliferation and type-2 cytokine production, regardless of the origin of NH cells ( Fig. 5a–d ). 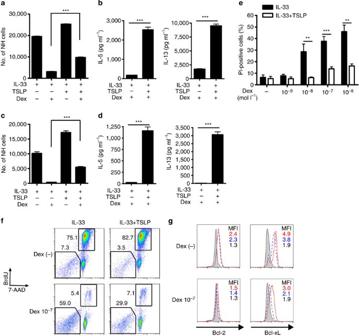Figure 5: TSLP inhibits corticosteroid-induced apoptosis of FALC and lung NH cells. (a–e) NH cells (5,000 cells per well) derived from FALC (a,b,e) or lungs (c,d) were cultured with IL-33 (10 ng ml−1) and/or TSLP (10 ng ml−1) in the presence or absence of dexamethasone (10−8;a–d, 10−9–10−6M;e) for 4 days. Number of propidium iodide (PI)-negative cells (a,c), concentrations of IL-5 and IL-13 in the culture supernatant (b,d), and the ratio of PI-positive cells among total cells (e) are presented. Mean±s.e.m.,n=3 for each group. **P<0.01, ***P<0.001 (Student’st-test). (f) Flow cytometric analysis of BrdU- and 7-AAD-stained FALC NH cells cultured with IL-33 (10 ng ml−1), TSLP (10 ng ml−1) with or without dexamethasone (10−7M) for 24 h. (g) Expression of Bcl-2 and Bcl-xL in FALC NH cells either unstimulated (filled area), stimulated with IL-33 (10 ng ml−1, dotted blue line) or stimulated with IL-33+TSLP (10 ng ml−1, solid red line). NH cells were cultured in the absence (upper panels) or presence (lower panels) of dexamethasone (10−7M). Data are representatives of three independent experiments. Figure 5: TSLP inhibits corticosteroid-induced apoptosis of FALC and lung NH cells. ( a – e ) NH cells (5,000 cells per well) derived from FALC ( a , b , e ) or lungs ( c , d ) were cultured with IL-33 (10 ng ml −1 ) and/or TSLP (10 ng ml −1 ) in the presence or absence of dexamethasone (10 −8 ; a – d , 10 −9 –10 −6 M; e ) for 4 days. Number of propidium iodide (PI)-negative cells ( a , c ), concentrations of IL-5 and IL-13 in the culture supernatant ( b , d ), and the ratio of PI-positive cells among total cells ( e ) are presented. Mean±s.e.m., n =3 for each group. ** P <0.01, *** P <0.001 (Student’s t -test). ( f ) Flow cytometric analysis of BrdU- and 7-AAD-stained FALC NH cells cultured with IL-33 (10 ng ml −1 ), TSLP (10 ng ml −1 ) with or without dexamethasone (10 −7 M) for 24 h. ( g ) Expression of Bcl-2 and Bcl-xL in FALC NH cells either unstimulated (filled area), stimulated with IL-33 (10 ng ml −1 , dotted blue line) or stimulated with IL-33+TSLP (10 ng ml −1 , solid red line). NH cells were cultured in the absence (upper panels) or presence (lower panels) of dexamethasone (10 −7 M). Data are representatives of three independent experiments. Full size image Although in cultures with IL-33 alone, the percentage of dead NH cells is increased by dexamethasone in a dose-dependent manner, dexamethasone (10 −9 –10 −6 M) fails to induce NH-cell death in the presence of TSLP ( Fig. 5e ). These results suggest that TSLP suppresses dexamethasone-induced apoptosis in NH cells. The fraction of cells in S phase in IL-33-stimulated NH cells, detected as a BrdU high 7-AAD high subset, is reduced by treatment with dexamethasone and this is not affected by addition of TSLP ( Fig. 5f ). In contrast, the fraction of NH cells in the BrdU low /7-AAD low subset, an indicative of apoptotic cells, is reduced in the IL-33+TSLP group compared with the cells treated with IL-33 alone ( Fig. 5f ), which is consistent with the results shown in Fig. 5e . Although IL-33+TSLP increases the expression of GATA3, a molecule essential for the differentiation and maintenance of group 2 ILC2s [28] , [29] , [30] including NH cells [30] , its expression is sensitive to corticosteroids ( Supplementary Fig. S11 ). We also evaluated the expression levels of the anti-apoptotic molecules, Bcl-2 and Bcl-xL and found that their expression is increased in NH cells cultured with IL-33 or IL-33+TSLP ( Fig. 5g , upper panels). Notably, the addition of TSLP preserves the expression of Bcl-xL even in dexamethasone-treated NH cells, while Bcl-2 expression is almost completely suppressed ( Fig. 5g , lower panels). STAT5 inhibitors attenuate corticosteroid resistance by TSLP To further examine the mechanisms of TSLP-induced corticosteroid resistance, we evaluated the TSLP signalling pathway in NH cells. We found that phosphorylation of STAT5 is increased in the nucleus of NH cells cultured with IL-33 and TSLP, but not with IL-33 alone, and this is not suppressed by dexamethasone ( Fig. 6a ). It has been reported that STAT5 binds to the glucocorticoid receptor and retains it the cytosol [31] . However, TSLP does not change the nuclear translocation/phosphorylation of glucocorticoid receptor in NH cells ( Fig. 6b ). 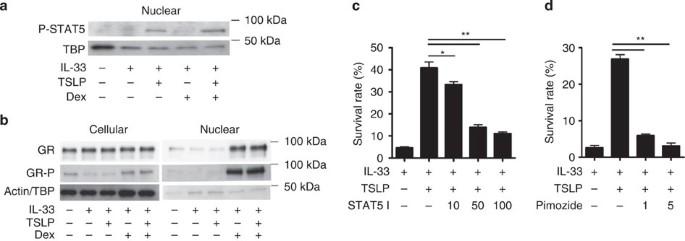Figure 6: STAT5 is the key molecule in TSLP-induced corticosteroid resistance. (a) Western blot analysis of phosphorylated STAT5 in the nucleus of FALC-derived NH cells cultured with IL-33 (10 ng ml−1), TSLP (10 ng ml−1), dexamethasone (10−8M) or their combination for 12 h. TATA-binding protein (TBP) is shown as a loading control. (b) Levels of total and phosphorylated glucocorticoid receptor (GR) in NH cells were assessed by western blot analysis. Actin and TBP were loading controls for cytoplasmic and nuclear components, respectively. (c,d) Survival rate (PI-negative cells/total cells) of NH cells cultured with IL-33 (10 ng ml−1), dexamethasone (Dex: 10−8M) and/or TSLP (10 ng ml−1) in the presence of a STAT5 inhibitor (c, compound 573108, 10–100 μM) or pimozide (d, 1 or 5 μM) for 4 days. Mean±s.e.m.,n=3 for each group. *P<0.05, **P<0.01 (ANOVA, Dunnet).P-values are presented as compared with IL-33+TSLP. Data are representatives of three independent experiments. Figure 6: STAT5 is the key molecule in TSLP-induced corticosteroid resistance. ( a ) Western blot analysis of phosphorylated STAT5 in the nucleus of FALC-derived NH cells cultured with IL-33 (10 ng ml −1 ), TSLP (10 ng ml −1 ), dexamethasone (10 −8 M) or their combination for 12 h. TATA-binding protein (TBP) is shown as a loading control. ( b ) Levels of total and phosphorylated glucocorticoid receptor (GR) in NH cells were assessed by western blot analysis. Actin and TBP were loading controls for cytoplasmic and nuclear components, respectively. ( c , d ) Survival rate (PI-negative cells/total cells) of NH cells cultured with IL-33 (10 ng ml −1 ), dexamethasone (Dex: 10 −8 M) and/or TSLP (10 ng ml −1 ) in the presence of a STAT5 inhibitor ( c , compound 573108, 10–100 μM) or pimozide ( d , 1 or 5 μM) for 4 days. Mean±s.e.m., n =3 for each group. * P <0.05, ** P <0.01 (ANOVA, Dunnet). P- values are presented as compared with IL-33+TSLP. Data are representatives of three independent experiments. Full size image A STAT5 inhibitor (compound 573108) counteracts the pro-survival effect of TSLP in a dose-dependent manner ( Fig. 6c ), suggesting that the inhibition of STAT5 impairs the TSLP-induced corticosteroid resistance of NH cells and NH-cell-mediated type-2 innate immune responses. A previous study has screened >1,000 pre-existing drugs and demonstrates that an anti-psychotic drug, pimozide, inhibits STAT5 (ref. 32 ). We found that a low dose (1 μM) of pimozide effectively counteracts the TSLP-induced resistance to corticosteroids of NH cells ( Fig. 6d ). The effects of TSLP in reducing the corticosteroid sensitivity of NH cells in vivo were further confirmed by co-administration of TSLP and IL-33 into the airways of mice ( Fig. 7a ). Although TSLP alone does not affect airway inflammation, co-administration of TSLP and IL-33 significantly increases the accumulation of eosinophils and NH cells, synthesis and release of IL-5 and IL-13, and mucin production in the epithelium and these processes are resistant to corticosteroid treatment ( Fig. 7b–f ). Oral administration of pimozide (1 mg kg −1 per day) effectively abrogates TSLP-induced corticosteroid resistance in vivo ( Fig. 7b–f ). These results indicate that the STAT5 pathway is critical for the acquisition of corticosteroid resistance. 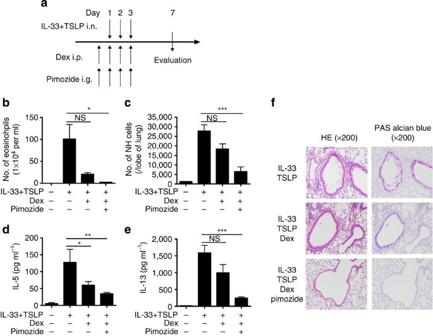Figure 7: Pimozide attenuates corticosteroid resistance in the IL-33 plus TSLP-induced asthma model. (a) Mice were treated with IL-33 (0.5 μg) and TSLP (0.1 μg) for 3 days, and dexamethasone (5 mg kg−1, intraperitoneally) and/or pimozide (1 mg kg−1, intragastrically) were administered at 24 and 1 h before IL-33+TSLP treatments. (b,c) Number of eosinophils in the BALF (b) and NH cells in the lung (c) 4 days after the final administration of IL-33 and TSLP. Mean±s.e.m.,n=3–6 for each group. NS, not significant. *P<0.05, **P<0.01, ***P<0.001 (ANOVA, Bonferroni). (d,e) Concentrations of IL-5 (d) and IL-13 (e) in the BALF were measured by ELISA. Mean±s.e.m.,n=3–6 for each group. NS, not significant. *P<0.05, **P<0.01, ***P<0.001 (ANOVA, Bonferroni). (f) Representative histology of the airways stained with hematoxylin and eosin (left panels) or periodic acid–Schiff (PAS)-alcian blue (right panels). Scale bar, 200 μm. Data are representatives of three independent experiments. Figure 7: Pimozide attenuates corticosteroid resistance in the IL-33 plus TSLP-induced asthma model. ( a ) Mice were treated with IL-33 (0.5 μg) and TSLP (0.1 μg) for 3 days, and dexamethasone (5 mg kg −1 , intraperitoneally) and/or pimozide (1 mg kg −1 , intragastrically) were administered at 24 and 1 h before IL-33+TSLP treatments. ( b , c ) Number of eosinophils in the BALF ( b ) and NH cells in the lung ( c ) 4 days after the final administration of IL-33 and TSLP. Mean±s.e.m., n =3–6 for each group. NS, not significant. * P <0.05, ** P <0.01, *** P <0.001 (ANOVA, Bonferroni). ( d , e ) Concentrations of IL-5 ( d ) and IL-13 ( e ) in the BALF were measured by ELISA. Mean±s.e.m., n =3–6 for each group. NS, not significant. * P <0.05, ** P <0.01, *** P <0.001 (ANOVA, Bonferroni). ( f ) Representative histology of the airways stained with hematoxylin and eosin (left panels) or periodic acid–Schiff (PAS)-alcian blue (right panels). Scale bar, 200 μm. Data are representatives of three independent experiments. Full size image Corticosteroid resistance is a major clinical problem in the treatment of asthma. The present study has demonstrated that, although by itself sensitive to corticosteroid, the IL-33/NH-cell pathway becomes resistant to corticosteroids in vitro and in vivo in the presence of TSLP and other STAT5-activating cytokines. TSLP is especially relevant to corticosteroid resistance in inflamed airways. Bronchial epithelial cells produce TSLP and the amounts of TSLP in the lung are significantly elevated in the asthmatic airways [22] , [26] , [27] . As shown here, the inhibition of TSLP or its key signalling molecule, STAT5, can restore the sensitivity of NH cells to corticosteroids. After we first reported NH cells in the FALC [10] , several groups have demonstrated the presence of similar group 2 ILCs in the lung and variously designated these cells as lung NH cells [15] , Lin − CD25 + CD44 hi lymphoid cells [33] or pulmonary ILC [16] . These lung-derived NH cells are present in Rag1 −/− mice, but deficient in Il7 −/− or Rag2 −/− Il2rg −/− mice [15] , [33] as are FALC NH cells [10] . In the present study, we also identified lung NH cells as Lin − Thy1 + c-Kit + Sca-1 + CD25 + IL-7R + ST2 dim cells. Compared with FALC NH cells, lung NH cells expressed lower amounts of ST2, although this pathway is still functional as lung NH cells proliferate and produce T H 2 cytokines in vitro in response to IL-33 alone. One previous study reported that lung NH cells require IL-2, IL-7 or TSLP for IL-33-induced proliferation [15] . The difference between their data and ours may be due to the different protocols employed for the isolation of lung NH cells; we used a combination of antibodies against Thy1, c-Kit and Sca-1, whereas the previous study used antibodies against Sca-1, c-Kit, IL-7R and CD25. The number of NH cells used in the proliferation assay may also be critical, because NH cells derived from FALC or lung do not proliferate well at a concentration of 1 × 10 3 cells per well or less, suggesting the presence of a NH-cell-derived paracrine factor(s) required for the effective proliferation of NH cells. Our data clearly demonstrate that IL-33-dependent proliferation and type-2 cytokine production in NH cells are blocked by corticosteroids in vivo and in vitro , which is in sharp contrast to IL-25-induced corticosteroid-resistant type-2 myeloid cells [23] . Corticosteroids suppress NH cells predominantly via the induction of apoptosis. However, NH cells become corticosteroid-resistant in the inflamed airways of the OVA+IL-33 model, suggesting the modification of corticosteroid sensitivity by the local inflammatory milieu. We identified IL-2, IL-7, IL-9 and TSLP as possible modifiers of NH-cell corticosteroid sensitivity in an in vitro assay. It has been reported that IL-2 (refs 34 , 35 ) and IL-7 (ref. 36 ) also induce corticosteroid resistance in T cells. Our data demonstrate that TSLP is also able to induce corticosteroid resistance in lymphoid-lineage cells. We confirmed the relevance of TSLP in corticosteroid resistance in airways inflamed by allergen exposure, as either TSLP inhibition with an antibody or genetic deficiency of TSLP abrogated corticosteroid resistance in mouse asthma models. This is relevant to clinical findings that levels of TSLP in airway epithelia and lamina propria are elevated in patients with severe [22] or fatal asthma [27] . TSLP expression can be induced in bronchial epithelial cells in response to various danger signals including protease antigens such as those of the house dust mite [37] . Furthermore, TSLP has an important role in T H 2-polarized allergen sensitization in the airways [26] . Our data suggest that this cytokine is also important for the modulation of the corticosteroid sensitivity in type-2 innate immune responses. TSLP-mediated corticosteroid resistance occurs more dominantly in NH cells than in T H 2 lymphocytes possibly due to the higher expression of TSLPR in NH cells. The receptors for IL-2, IL-7 and IL-9 share a common-γ chain [38] , and TSLP and IL-7 receptors share IL-7R [39] , all of which activate a STAT5 signalling pathway [38] . We found that the activation of STAT5 cannot be suppressed by corticosteroids in NH cells. Therefore, it is reasonable to speculate that the induction of the STAT5 pathway by TSLP and common-γ chain family cytokines is related to the corticosteroid resistance in NH cells. In CD4 T lymphocytes, the activation of STAT5 by IL-7 upregulates Bcl-2 and Bcl-xL, protecting the cells from apoptosis [40] . Similarly, TSLP decreased the apoptosis of NH cells with a concomitant induction of Bcl-xL and the induction of Bcl-xL was resistant to corticosteroids. In addition, STAT5 inhibitors reverse the effects of TSLP on the corticosteroid-resistant survival of NH cells. Another possible mechanism by which STAT5 induces corticosteroid resistance is the formation of a complex with glucocorticoid receptors thus inhibiting their nuclear translocation [30] . However, TSLP did not change the nuclear translocation or the phosphorylation of glucocorticoid receptor in NH cells. Our data collectively suggest that drugs targeting either TSLP or STAT5 may be efficacious for the management of patients with corticosteroid-resistant asthma. Anti-TSLP antibodies are under development for use as anti-asthma drugs. Although currently available STAT5 inhibitors are too toxic for clinical use, ‘drug repositioning’ research, which examines newly identified pharmacological activities of previously established drugs for use in different therapeutic indications [41] , identified pimozide, an anti-psychotic drug, as a potent inhibitor of STAT5 (ref. 32 ). As the safety of this drug is already established, it is now under development for the treatment of imatinib-resistant chronic myeloid leukemia [32] . Our data suggest that a low concentration (1 μM) of pimozide in vitro and a low-dose (1 mg kg −1 per day) in vivo exhibit synergistic effects with corticosteroids on NH cells and therefore the clinical use of this drug may be feasible for the treatment of corticosteroid-resistant asthma. In conclusion, the corticosteroid sensitivity of the IL-33/NH-cell pathway is modified by epithelium-derived cytokines such as TSLP. These data suggest that, in the conditions in which IL-33 and NH cells have a crucial role in its pathophysiology, for example, severe asthma or its exacerbation complicated with fungal sensitization/colonization or viral infection, anti-TSLP or anti-STAT5 drugs such as pimozide can provide a new therapeutic approach to overcome corticosteroid resistance. Mice Six- to eight-week-old male C57BL/6 mice were purchased from Japan SLC (Tokyo, Japan) and maintained in a pathogen-free environment at Keio University or RIKEN Center for Integrative Medical Sciences (RIKEN-IMS). Tslpr −/− mice [42] were provided by Susumu Nakae of the University of Tokyo. All animal experiments and handling procedures were approved by the Keio University and RIKEN-IMS Animal Care and Use Committees and were performed in accordance with institutional guidelines. Antibodies Anti-Bcl-2 antibody (C-2) was obtained from Santa Cruz Biotechnology (Santa Cruz, CA, USA). Anti-Bcl-xL (54H6), anti-phospho-STAT5 (Tyr694, D47E7) and anti-TBP antibodies were obtained from Cell Signaling Technology (Danvers, MA, USA). Anti-TSLP antibody, anti-IL-7 antibody and goat IgG isotype control antibody were from R&D systems (Minneapolis, MN, USA). Biotin-conjugated anti-CD4 (GK1.5), anti-CD8α (53-6.7), anti-CD11c (HL3), anti-CD11b (M1/70), anti-CD19 (1D3), anti-NK1.1 (PK136), anti-Gr-1 (RB6-8C5), anti-TER119, anti-B220 (RA3-6B2), Pacific blue-conjugated anti-Sca-1 (E13-161), PerCP Cy5.5-conjugated anti-CD25 (PC61), PE-conjugated anti-Thy1.2 (53-2.1), APC Cy7-conjugated anti-streptavidin, anti-IL-2 antibody (S4B6) and Rat IgG2a isotype control antibody were from BD Pharmingen (San Diego, CA, USA). PECy7-conjugated c-Kit (2B8), biotin-conjugated anti-FcεRI (MAR-1), PE-conjugated anti-IL-5 (TRFK5), APC-conjugated anti-IL-13 (eBio13A) and APC-conjugated anti-IL-7R (A7R34) were from eBioscience (La Jolla, CA, USA). FITC-conjugated anti-T1/ST2 was from MD Bioscience (St Paul, MN, USA). Anti-IL-17RB was kindly provided by Hiroshi Watarai and anti-CD16/CD32 (2.4G2) was purified from supernatant. Antibody dilutions used in this study are listed in Supplementary Table S1 . Compounds and cytokines Pimozide and dexamethasone were obtained from Sigma (St Louis, MO, USA) and a STAT5 inhibitor (573108) from Calbiochem (San Diego, CA, USA). Recombinant mouse cytokines including IL-2, IL-15, IL-18, IL-21, IL-23, IL-25, IL-27, IL-33, TSLP and TNF-α were from R&D systems. IL-3, IL-5, IL-6, IL-7, IL-9 and IL-12 were from PeproTech (Rocky Hill, NJ, USA). Induction of asthma and treatment in a mouse model Recombinant mouse IL-33 (0.1–1 μg) and/or TSLP (0.1 μg) in 40 μl PBS was administered intranasally to mice anesthetized with ketamine. For the asthma model, mice were sensitized by intraperitoneal injections of OVA (15 μg) with alum on day 0, 7, 15 and then were challenged with intranasal administration of OVA (10 ng) in 40 μl PBS on days 22–24. Dexamethasone (0.5–5 mg kg −1 ) was administered i.p. at 24 and 1 h before the nasal challenge of IL-33/OVA/TSLP. Neutralizing antibodies (25 μg) against TSLP, IL-2 or IL-7, or isotype control antibodies were administered intranasally, and pimozide (1 mg kg −1 ) diluted with 0.1% hydroxypropyl methylcellulose was administered intragastrically at the same time as dexamethasone. Four days after the final challenge with IL-33/OVA/TSLP, mice were killed by pentobarbital overdose. BALF was obtained by flushing the lungs with 0.7 ml PBS via tracheal cannulae. The cell counts in the lavage fluids were determined with a hemocytometer, and differential cell counts were determined in cytospin preparations stained with Diff-Quick (Symex, Kobe, Japan); >200 cells were analysed using conventional morphologic criteria. The supernatants were collected and stored at −80 °C for cytokine assays. The left lung lobes were fixed in 4% formaldehyde and stained with hematoxylin and eosin or periodic acid–Schiff-Alcian blue for histological analyses. The right upper lobes of the lungs were processed for analysis of lung NH cells, and the remaining lung tissues were homogenized for cytokine assays and RNA isolation. Analyses and isolation of NH cells To isolate NH cells, C57BL/6 female retired breeder mice (>4 month old) were used. Lungs were minced and digested with Liberase-TM (Roche, Tokyo, Japan) and DNase (Warthington, Lakewood, NJ, USA) for 1 h at 37 °C, then mashed through 40 μm cell strainers to obtain single-cell suspension. The cells were stained with biotin-conjugated antibody mixtures for lineage markers (CD4, CD5, CD8, CD11c, CD11b, CD19, NK1.1, Gr-1, TER119, FcεRI and B220), Pacific blue-conjugated anti-Sca-1, PECy7-conjugated c-Kit (CD117), APC-conjugated anti-IL-7Rα (CD127), FITC-conjugated anti-T1/ST2, PerCPCy5.5-conjugated anti-CD25, PE-conjugated anti-Thy1.2 and APCCy7-conjugated anti-streptavidin, and analysed using a FACS AriaIIu (BD Biosystems, San Jose, CA, USA). Lin − Sca-1 + c-Kit + IL-7R + CD25 + ST2 dim cells were counted as lung NH cells. Lung NH cells were isolated for in vitro studies as a cell fraction of Lin − Sca-1 + c-Kit + Thy1 + cells. To isolate NH cells from FALC, mesenteries were separated from intestine and mesenteric lymph nodes removed. Materials were then digested with collagenase as previously reported [10] . NH cells were isolated as Lin − Sca-1 + c-Kit + cells by cell sorting. All data were analysed by FlowJo (TreeStar, Ashland, OR, USA). Proliferation and cytokine production assays of NH cells Purified NH cells were cultured at a density of 5,000 cells per well in 96-well round bottom plates in 200 μl RPMI-1640 media containing 10% FCS, HEPES buffer, non-essential amino acids, penicillin, streptomycin and 2-mercaptoethanol at 37 °C for 4 days. To evaluate the effect of various cytokines, IL-2, IL-3, IL-5, IL-6, IL-7, IL-9, IL-12, IL-15, IL-18, IL-21, IL-23, IL-25, IL-27, IL-33, TSLP and TNF-α were added to the culture medium at a final concentration of 10 ng ml −1 with or without dexamethasone (10 −9 –10 −6 M), a STAT5 inhibitor (compound 573108, 10–100 μM) and/or pimozide (1 or 5 μM). One hundred microliter of supernatants were collected for the cytokine assay, and NH cells were stained by propidium iodide to count live cells by flow cytometry. Intracellular staining of NH cells with BrdU and 7-aminoactinomycin D (7-AAD) were also performed according to the manufacturer’s protocols (BrdU Flow Kit, BD Pharmingen), and then analysed with flow cytometry. ELISAs Amounts of IL-5 and IL-13 in BALF and in culture supernatants and amounts of TSLP in the supernatants of lung homogenates were measured by Quantikine ELISA kits (R&D Systems) according to the manufacturer’s protocol. RNA isolation and real-time quantitative PCR RNA was isolated from lung homogenates with RNeasy mini kits according to the manufacturer’s instructions (Qiagen, Tokyo, Japan) and cDNA was generated with SuperScript reverse transcriptase (Invitrogen, Carlsbad, CA, USA). The expression levels of IL-33 (5′- ATGAGACCTAGAATGAAGTATTC -3′, 5′- GCACAGGCGTTTTACTGCATT -3′), IL-2Rα (5′- AGGAGAGGGCTTTGAATGTG -3′ 5′- TTGCTGATGTTGGGGTTTCT -3′), IL-7Rα (5′- CATTTCACTCGTAAAAGAGCCC -3′ 5′- TGGAAGTGGATGGAAGTCAA -3′), TSLPR (5′- ACTGTGACATCACCCCGTG -3′, 5′- GACATGGCATGGGCACTC -3′) and TSLP (5′- GCCATTTCCTGAGTACCGTC -3′, 5′- TTCACTCCCCGACAAAACAT -3′) were measured by real-time quantitative PCR using SYBR Green Master Mix (Applied Biosystems, FosterCity, LA, USA) and an ABI7500 real-time PCR system (Applied Biosystems). Intracellular flow cytometric analyses NH cells were cultured with IL-33 (10 ng ml −1 ), TSLP (10 ng ml −1 ) and/or dexamethasone (10 −7 M) for 24 h and intracellular staining using IntraPrep (Beckman Coulter, Marseille, France) was performed with a mouse anti-Bcl-2 antibody or a rat anti-Bcl-xL antibody and FITC-conjugated anti-mouse IgG antibody and rat IgG antibody, respectively. Cells were then analysed by flow cytometry. Lung cells were stimulated for 3 h with PMA (30 ng ml −1 ; Sigma), ionomycin (500 ng ml −1 ; Calbiochem, San Diego, CA, USA) and brefeldin A at the recommended concentrations (eBioscience). Cells were then stained intracellularly with PE-conjugated anti-IL-5 and APC-conjugated anti-IL-13. CD4 T cells identified as CD3 + CD4 + cells and NH cells were analysed by flow cytometry. Measurement of airway hyperresponsiveness Four days after the final challenge, mice were anesthetized using ketamine and airway hyperresponsiveness were measured by FlexiVent system (SCIREQ, Canada) using methacholine (25–100 mg ml −1 ). Generation of bone marrow chimeric mice Equal number of bone marrow cells from wild-type (WT, CD45.1) and Tslpr −/− (CD45.2) mice were mixed and transferred into WT (CD45.1 × CD45.2) mice after 6 Gy irradiation. As a control, equal number of bone marrow cells from WT (CD45.1) and WT (CD45.2) mice were mixed and transferred. Western blot analyses NH cells were cultured with IL-33 (10 ng ml −1 )±TSLP (10 ng ml −1 )±dexamethasone (10 −7 M) for 12 h, and nuclear and cytoplasmic extracts were prepared with NE-PER Nuclear and Cytoplasmic Extraction Reagents Kits (Pierce, Yokohama, Japan). Lysates were run on gels and blotted with anti-phosphorylated STAT5 antibody (Cell Signaling Technology). To control the quality of nuclear and cytoplasmic proteins, anti-TATA-binding protein (TBP) and anti-actin antibodies were used, respectively. Statistics All data are presented as means±s.e. Data were analysed with GraphPad Prism 4 (GraphPad Software). The Student’s t -test was used to determine statistical significance between two groups. One-way ANOVA with Bonferroni adjustment or a Dunnet test were used for the comparison of more than three groups. All reported P- values were based on two-sided tests. How to cite this article: Kabata, H. et al . Thymic stromal lymphopoietin induces corticosteroid resistance in natural helper cells during airway inflammation. Nat. Commun. 4:2675 doi: 10.1038/ncomms3675 (2013).